ReducingMSH4copy number prevents meiotic crossovers between non-homologous chromosomes inBrassica napus In allopolyploids, correct chromosome segregation requires suppression of non-homologous crossovers while levels of homologous crossovers are ensured. To date, no mechanism able to specifically inhibit non-homologous crossovers has been described in allopolyploids other than in bread wheat. Here, we show that reducing the number of functional copies of MSH4 , an essential gene for the main crossover pathway, prevents non-homologous crossovers in allotetraploid Brassica napus . We show that non-homologous crossovers originate almost exclusively from the MSH4 -dependent recombination pathway and that their numbers decrease when MSH4 returns to single copy in B. napus ; by contrast, homologous crossovers remain unaffected by MSH4 duplicate loss. We also demonstrate that MSH4 systematically returns to single copy following numerous independent polyploidy events, a pattern that is probably not by chance. These results suggest that stabilization of allopolyploid meiosis can be enhanced by loss of a key meiotic recombination gene. Polyploidy (Whole-Genome Duplication, WGD) has played a pervasive role in the evolution of many living organisms [1] . Many eukaryotes descend from polyploid ancestors that experienced massive duplicate gene loss over millions of years and ultimately reverted to a diploid state [1] . The long-term survival of newly formed polyploids depends, however, on their ability to withstand the extensive genomic instability that accompanies the onset of polyploid formation. Most notably, nascent allopolyploids, which result from interspecific hybridization followed by WGDs, require meiotic adaptation to safeguard genome stability and fertility; otherwise, crossover formation between the chromosomes inherited from the allopolyploid’s progenitors (i.e. the homoeologues) will disrupt chromosome segregation and result in the production of aneuploid gametes [2] , [3] . Stabilization of allopolyploid meiosis thus requires that inter-homoeologue crossover formation is prevented while levels of homologous crossovers are ensured. How meiosis has adapted to cope with allopolyploidy has only been deciphered in allohexaploid wheat, where a duplication of the ZIP4 gene within the Ph1 locus prevents maturation of crossovers between non-homologous chromosomes [4] , [5] , [6] , [7] . ZIP4 is an essential factor for the main crossover pathway [8] , [9] (called the class I or ZMM pathway) that also includes a set of other critical proteins (e.g., MER3, MSH4, MSH5, SHOC1, HEI10, PTD) in plants. While there are numerous examples of allopolyploids that have adapted meiosis to prevent homoeologous crossovers, no other gene has been identified that influences the rate of homoeologous recombination in allopolyploids. In a previous paper [10] , we proposed that meiotic adaptation in established polyploids could involve ‘fine-tuning’ the progression or the effectiveness of meiotic recombination. One potential pathway to “fine-tune” meiosis in newly-formed polyploids is through gene loss. This process has recently gained attention as a driver of functional innovation [11] , [12] and massively affects the evolution of recent polyploid genomes in a process referred to as fractionation [13] . Genes involved in meiotic recombination (and DNA repair in general [14] , [15] ) seem especially susceptible to fractionation as they tend to return to a single copy more rapidly than genome average following subsequent and/or independent duplications [10] . In this paper, we ask whether the loss of some meiotic recombination gene duplicates can contribute to improved meiosis in these organisms. To address this question, we first re-evaluate the patterns of duplicate gene loss and retention for different genes encoding proteins from the class I crossover pathway. We then describe how copy number reduction of MSH4 (the ZMM gene that shows the most rapid fractionation) affects crossover formation in an allopolyploid ( Brassica napus ) to potentially enhance meiosis. Brassica napus (AACC, 2n = 38) is a recent allotetraploid crop bred for high seed yield, that originated from interspecific hybridizations between the ancestors of B. rapa (AA, 2n = 20) and B. oleracea (CC, 2n = 18) ~7500 years ago [16] . It is also, and most importantly, one of only two allopolyploid species (along with bread wheat [5] , [6] , [7] ) for which meiosis has been thoroughly analyzed [17] . We focused on crossover formation between both homologous and homoeologous chromosomes; the latter, which are rare events in euploids (AACC), are readily quantifiable in allohaploid plants obtained by microspore culture [17] . These plants only contain one unique copy of each chromosome (AC, n = 19) so that (almost) all crossovers observed in allohaploids involve homoeologues. Here, we show that regular meiosis is achieved in B. napus even when the number of functional MSH4 copies is reduced to a minimum. By contrast, we demonstrate that the number of crossovers formed between homoeologues responds to MSH4 dosage. This indicates that loss of one MSH4 copy has no negative impacts and is potentially beneficial for B. napus meiosis, which improves when crossovers between homoeologues are suppressed. Convergent loss of duplicated recombination genes post-WGDs Building on previous work [10] , we first measured the extent to which gene duplicates encoding plant ZMM proteins were lost or retained following >40 independent plant WGDs ranging in age from few thousand to more than 150 million years. Four ZMM s show a conspicuous pattern of rapid duplicate gene loss following WGDs (Fig. 1 ; Supplementary Figs. 1 – 3 ) with a single gene encoding MER3, MSH4, MSH5 and ZIP4 proteins in almost all angiosperms other than the most recent polyploids (i.e., those that formed <10,000 years ago). In paleopolyploids that have returned to a diploid state post-WGD, the presence of duplicates for these four ZMM remains an exception usually limited to those with the next most recent WGDs: e.g., MSH5 in Glycine max (5–9 million years old WGD [18] ); MER3 and ZIP4 in Linum usitatissimum (5–13 million years old WGD [19] ) (Fig. 1 ; Supplementary Figs. 1 – 3 ). By contrast, a slightly higher number of duplicates is observed among the genes encoding SHOC1, PTD and, most importantly, HEI10 (Fig. 1 ; Supplementary Figs. 4 – 6 ). Fig. 1 ZMM gene copy numbers in angiosperms. a Bar charts indicating the number of angiosperms showing one to six complete copies of the genes encoding each ZMM protein. Partial/fractionated copies are excluded. The different charts are based on a number of species ranging from 79 (MSH5) to 87 (HEI10). b Sector chart showing the age of the retained duplicates, as estimated by the age of the WGD they originate from. Only complete copies are considered here. Duplicates generated by small scale duplications (SSD) and/or that could not be associated with a specific WGD event are indicated in grey (i.e., age not specifically defined). c Maximum likelihood trees based on MSH4 amino acid sequences. For the sake of clarity, species names are indicated instead of gene names. Coloured disks superimposed along the branches of the tree give the age range for past WGDs (i.e., dark orange: 7000 years to 1 MY; light orange: 1 to 20 MY; light green: 20 to 50 MY; light blue: 50 to 85 MY; dark blue: 85 to 125 MY; violet: more than 125 MY). Full-length duplicates/triplicates (marked by solid arrows) and duplicates with one fractionated copies (marked by open arrows) are written with the colour that corresponds to the age of the WGD. Duplicates originating from SSD are written in magenta. Regarding the most recent WGD (i.e., dark orange: 7000 years to 1 MY), only allopolyploids are represented because there is no way to account for the presence of MSH4 “duplicates” in extant autopolyploids, which truly correspond to (multiple) real alleles. The connectors superimposed over the phylogeny associates the full-length and fractionated copies of MSH4 in Populus trichocarpa Full size image The most striking example of precipitous ZMM duplicate loss is MSH4 , which shows only one intact copy in all diploid species (Fig. 1 ). To determine whether rapid MSH4 duplicate loss post-WGD is specific to angiosperms, we expanded our analysis to include a taxonomically broad set of 95 fungi and 39 animal species that encompass 12 additional WGDs ranging in age from few thousand to almost 500 million years (Supplementary Figs. 7 – 8 ). Again, we identified only one intact copy of MSH4 in all species except the very recent polyploids ( Zygosaccharomyces rouxii ) and Diplocarpon rosae and Hortaea werneckii , two fungi that have retained 80 and 95% of gene duplicates post-WGDs, respectively [20] , [21] (Supplementary Fig. 8 ). Remnants of a second copy of MSH4 carrying inactivating changes were detected in only three plant ( L. usitatissimum , G. max and Populus trichocarpa ; Fig. 1c ) and two animal ( Salmo salar and Oncorhynchus mykiss ; Supplementary Fig. 7 ) species. The inactivating changes found (important sequence gaps, mutations and truncations in exonic sequences) in these MSH4 pseudogenes, are likely signatures of ongoing fractionation. B. napus carries two differentially expressed copies of MSH4 The results above demonstrate that MSH4 is a textbook case of the rapid loss of meiotic recombination duplicates following WGDs; they also indicate that, although very rapid on an evolutionary timescale (i.e., a few million years), MSH4 -duplicate loss is not immediate. As shown in Fig. 1 , B. napus contains two full-length MSH4 homologues, hereafter referred as to BnaA.MSH4 (marked as Brassica napus homoeo2 on Fig. 1 ) and BnaC.MSH4 (marked as Brassica napus homoeo1 on Fig. 1 ). These two copies correspond to homoeologues sensu [22] . A partial (4 exons instead of 24) copy of MSH4 was also found tandemly arrayed with BnaA.MSH4 (Fig. 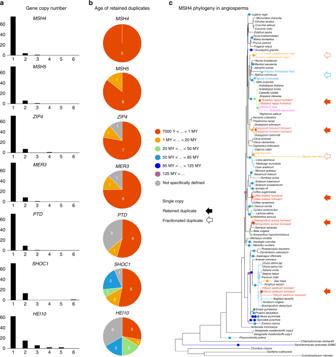Fig. 1 ZMMgene copy numbers in angiosperms.aBar charts indicating the number of angiosperms showing one to six complete copies of the genes encoding each ZMM protein. Partial/fractionated copies are excluded. The different charts are based on a number of species ranging from 79 (MSH5) to 87 (HEI10).bSector chart showing the age of the retained duplicates, as estimated by the age of the WGD they originate from. Only complete copies are considered here. Duplicates generated by small scale duplications (SSD) and/or that could not be associated with a specific WGD event are indicated in grey (i.e., age not specifically defined).cMaximum likelihood trees based on MSH4 amino acid sequences. For the sake of clarity, species names are indicated instead of gene names. Coloured disks superimposed along the branches of the tree give the age range for past WGDs (i.e., dark orange: 7000 years to 1 MY; light orange: 1 to 20 MY; light green: 20 to 50 MY; light blue: 50 to 85 MY; dark blue: 85 to 125 MY; violet: more than 125 MY). Full-length duplicates/triplicates (marked by solid arrows) and duplicates with one fractionated copies (marked by open arrows) are written with the colour that corresponds to the age of the WGD. Duplicates originating from SSD are written in magenta. Regarding the most recent WGD (i.e., dark orange: 7000 years to 1 MY), only allopolyploids are represented because there is no way to account for the presence ofMSH4“duplicates” in extant autopolyploids, which truly correspond to (multiple) real alleles. The connectors superimposed over the phylogeny associates the full-length and fractionated copies ofMSH4inPopulus trichocarpa 1 ; Supplementary Table 1 ). This additional copy is not transcribed during meiosis (based on B. napus meiotic RNAseq [23] ) and was therefore not considered for further analyses. 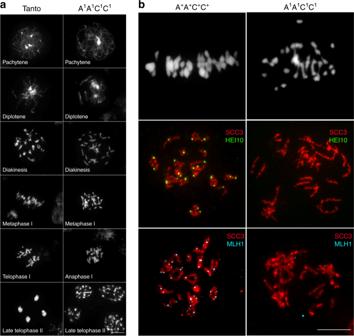Fig. 2 Meiotic progression and crossover formation in presence and absence of functional MSH4.aComparative DAPI staining of wild type (B. napuscvTanto) andA1A1C1C1msh4double mutant. Different meiotic stages are illustrated: pachytene, diplotene, diakinesis metaphase I, Anaphase/telophase I, Late anaphase II, scale bar 10 µm.bChiasmata and immunolabeled class I COs in WT andA1A1C1C1msh4double mutant. The upper pictures show DAPI spreads of metaphase I. The middle pictures show dual immunolocalization of SCC3 and HEI10 at diakinesis stage. The lower pictures show dual immunolocalization of SCC3 and MLH1. Scale bar 10 µm We observed that BnaA.MSH4 and BnaC.MSH4 are both transcribed during male meiosis in the three varieties analyzed, with BnaC.MSH4 contributing most to MSH4 expression in B.napus ; in all varieties, the balance between A/C contribution was in the range of 1/6 to 1/3 (Supplementary Table 2 ). This feature is unique to MSH4 (compared to MSH5 , MER3 and ZIP4 ) and offers more opportunities to assess the effect of varied ZMM dosage on crossover formation (see below). We, therefore, focused on this gene  for further analyses. The predicted amino acid sequences of BnaA.MSH4 and BnaC.MSH4 , consolidated using B. napus meiotic RNAseq data [23] , both contained canonical MutS domains including the highly conserved C-terminal MutSac domain, which is essential for ATPase and DNA-binding activities [24] (Supplementary Fig. 9 ). We identified and selected using TILLING (Supplementary Fig. 10 ) one mutant allele in BnaA.MSH4 (hereinafter referred as to bnaA.msh4-1 , symbolized by A 1 ) and two mutant alleles in BnaC.MSH4 (hereinafter referred as to bnaC.msh4-1 , symbolized by C 1 , and bnaC.msh4-2 , symbolized by C 2 , respectively). These alleles were the only ones for which the conserved MutSac domain was disrupted by early stop codons introduced by a point-nonsense mutation ( bnaC.msh4-1 ) or because of splice site mutations ( bnaA.msh4-1 and bnaC.msh4-2 ) (Supplementary Fig. 11 ). Homologous crossovers largely depend on MSH4 in B. napus To ensure that the identified mutations did indeed compromise MSH4 function, we first assessed whether plants carrying only msh4 mutant alleles ( A 1 A 1 C 1 C 1 and A 1 A 1 C 2 C 2 : Supplementary Fig. 12 ) showed a severe reduction in crossover leading to the occurrence of numerous univalents (i.e. chromosome that failed to form crossovers) at metaphase I [25] , [26] . We first analyzed the progression of male meiosis in WT B. napus cv. Tanto , the accession in which msh4 mutations were identified. Our cytological survey showed that meiosis was very regular in cv. Tanto , like in other B. napus accessions [17] . During prophase I, meiotic chromosomes condensed, recombined and underwent synapsis, the close association of two homologous chromosomes via the Synaptonemal Complex (SC), which was complete at pachytene. From diakinesis to metaphase I, 19 discrete bivalents were identifiable in all cells (Fig. 2a ). They consisted of pairs of homologous chromosomes bound together by chiasmata, the cytological manifestation of meiotic crossovers. We estimated that 57% of the bivalents in WT were rings with both arms bound by chiasmata while the remaining 43% were rods with only one arm bound by chiasmata. Assuming that rod and ring bivalents had only one and two crossovers, respectively, we estimated a mean of 30.0 chiasmata per cell in A + A + C + C + ( n = 28; Fig. 2 , Table 1 ). This could be an underestimate, however, given that it is not possible to distinguish cytologically single from multiple crossovers clustered on a single arm. The second meiotic division then took place and produced balanced tetrads of four microspores (Late telophase in Fig. 2a ). Fig. 2 Meiotic progression and crossover formation in presence and absence of functional MSH4. a Comparative DAPI staining of wild type ( B. napus cv Tanto ) and A 1 A 1 C 1 C 1 msh4 double mutant. Different meiotic stages are illustrated: pachytene, diplotene, diakinesis metaphase I, Anaphase/telophase I, Late anaphase II, scale bar 10 µm. b Chiasmata and immunolabeled class I COs in WT and A 1 A 1 C 1 C 1 msh4 double mutant. The upper pictures show DAPI spreads of metaphase I. The middle pictures show dual immunolocalization of SCC3 and HEI10 at diakinesis stage. The lower pictures show dual immunolocalization of SCC3 and MLH1. Scale bar 10 µm Full size image Table 1 Crossover reduction in euploid and allohaploid B. napus msh4 mutants Full size table In the A 1 A 1 C 1 C 1 and A 1 A 1 C 2 C 2 double mutants, the early stages of prophase I were similar to those of WT B. napus cv. Tanto (Fig. 2a ). We confirmed that synapsis was complete in these plants, as demonstrated by immunolocalization of ZYP1 protein, a major component of the central element of the SC [27] (Supplementary Fig. 13 ). Meiotic defects became obvious at the end of meiotic prophase when the bivalent formation was strongly compromised in both A 1 A 1 C 1 C 1 and A 1 A 1 C 2 C 2 (see metaphase I in Fig. 2a , b and Supplementary Fig. 14 ). We observed a mean number of 20.4 univalents (53% of chromosomes) that coexisted with 8.8 bivalents in A 1 A 1 C 1 C 1 (Table 1 ). Contrary to WT, the majority of bivalents were rods (84%). At metaphase I, the reduction in chiasmata frequency was thus very evident, dropping down to an average of 9.9 chiasmata per cell (Table 1 ). The univalents then segregated randomly, resulting in unbalanced tetrads (See late telophase II in Fig. 2a ). To test whether the msh4 mutant alleles completely suppress MSH4 activity, we immuno-localized HEI10 and MLH1, two proteins that specifically mark the sites of MSH4-dependent (i.e., class I) crossovers at diakinesis [28] . We consistently counted 29 foci for the HEI10 and MLH1 proteins (Table 1 ; Figs. 2 , 3 ) in the A + A + C + C + plants that only carries WT MSH4 alleles but is sibling to A 1 A 1 C 1 C 1 . By contrast, in the A 1 A 1 C 1 C 1 and A 1 A 1 C 2 C 2 double mutants, the residual chiasmata observed were not marked by HEI10 or MLH1 foci (Table 1 ; Fig. 2b and Supplementary Fig. 14 ), suggesting the absence of class I crossovers in these plants. This indicated that A 1 A 1 C 1 C 1 and A 1 A 1 C 2 C 2 were null msh4 mutants and that bnaA.msh4-1 , bnaC.msh4-1 and bnaC.msh4-2 alleles encoded nonfunctional MSH4 proteins. Fig. 3 Robustness of ZMM-dependent crossovers to MSH4 copy number reduction in B. napus euploids. Scatter plot of HEI10 (class I crossover) foci in the different genotypes, as determined by HEI10 immunolocalization. *** indicates highly significant variations ( p -value < 0.0001) according to Kruskal–Wallis test. Error bars show standard deviation. Means (black bar) are also indicated Full size image Total crossover numbers are unaffected by MSH4 copy number To examine the functional consequences of loss of MSH4 copies, we characterized the meiotic behaviour of plants carrying different combinations of WT and mutant alleles (Supplementary Fig. 12 ). We verified beforehand that loss of one copy is not compensated by a transcriptional upregulation of the remaining MSH4 WT alleles, a rare but not unheard phenomenon [29] , [30] , [31] . The relative contribution of BnaA.MSH4 and BnaC.MSH4 along with their summed expression suggested no obvious decay or transcriptional compensation between functional and mutant msh4 alleles (Supplementary Fig. 15 ). We then moved on to the cytological survey of the exact same plants. We observed that functional loss of BnaA.MSH4 , the least expressed MSH4 copy, or BnaC.MSH4 , the most expressed MSH4 copy, all resulted in a WT-like meiosis (Fig. 3 ; Supplementary Figs. 16 and 17 ). The A 1 A 1 C + C + , A + A + C 1 C 1 and A + A + C 2 C 2 plants all showed 19 bivalents at metaphase I (Supplementary Fig. 16 ) and the same number of HEI10 foci as the WT (Fig. 3 ; Supplementary Fig. 17 ). These results indicated that, irrespective of their unequal transcriptional contribution, BnaA.MSH4 and BnaC.MSH4 are both equally functional and able to complement one another. We then explored the extreme situation where BnaC.MSH4 was completely depleted while only one allele of the BnaA.MSH4 was functional. This plant, i.e., A + A 1 C 1 C 1 , carried the minimum functional MSH4 dosage possible, with only one functional allele of the least expressed copy (e.g., >90% reduction in functional transcript). Despite this minimal composition, A + A 1 C 1 C 1 showed the exclusive bivalent configuration and about 31 HEI10 foci per meiocyte as in WT (Fig. 3 ; Supplementary Figs. 16 f and 17f ). All these results indicated that normal class I crossover formation is not sensitive to MSH4 duplicate loss, providing that (at least) one functional copy of MSH4 is present in the plant. Homoeologous crossovers are affected by MSH4 copy number We then focused on crossover formation between homoeologous chromosomes in allohaploid plants produced from the two F1 hybrids ( A + A 1 C + C 1 and A + A 1 C + C 2 ; Supplementary Fig. 12 ). As in euploids, we first verified that there was no transcriptional compensation between functional and mutant MSH4 alleles in allohaploids showing varied number and assortments of WT (A + or C + ) and mutant msh4 alleles (A 1 , C 1 or C 2 ) (Supplementary Fig. 15 ). We then estimated that WT allohaploids ( A + C + ) showed on average 6.3 chiasmata distributed over a mean number of 1 ring and 4.4 rod bivalents (Fig. 4 and Table 1 ). Interestingly, we observed a slight but significant decrease in chiasmata frequency (compared to WT allohaploids t > 4.3, p -value < 0.0001, according to t -test) when the least expressed copy was depleted; the mean number of chiasmata in A 1 C + plants dropped down to 5.1 crossovers (Fig. 4 ; Table 1 ). A stronger and significant reduction in chiasmata was observed when the most expressed copy was depleted, down to 2.2 chiasmata per cell in A + C 1 (compared to A 1 C + ; t > 8.5, p -value < 0.0001, according to t -test) and 2.7 chiasmata per cell in A + C 2 (compared to A 1 C + ; t > 2.4, p -value < 0.02, according to t -test) allohaploids, respectively (Fig. 4 ; Table 1 ). In these two plants, almost all bivalents were rods and only very rare ring bivalents were observed. Finally, when both MSH4 copies were depleted, the number of residual chiasmata was further decreased, down to 0.7 in A 1 C 1 (compared to A + C 1 ; t > 5.4, p -value < 0.0001, according to t -test) and 1.3 in A 1 C 2 (Fig. 4 and Table 1 ). Contrary to the euploids, immunolocalization of MLH1 and HEI10 proteins could not be used to confirm the decay of class I crossovers in all these plants. We have previously shown that in B. napus allohaploid meiosis the two proteins do not always co‐localize during meiosis in B. napus allohaploid [17] , which makes Class I CO estimates technically impossible. This notwithstanding, our results indicated that inter-homoeologue class I crossover formation is sensitive to MSH4 duplicate loss (Fig. 4 ). Fig. 4 Decreased crossovers upon MSH4 copy number reduction in B. napus allohaploids. Scatter plot showing the number of chiasmata estimated for allohaploids carrying varying doses of functional and msh4 mutant alleles. Each genotype is illustrated below with a cytological image as example. N.s indicates non-significant variations whereas *** indicates highly significant variations ( p -value < 0.0001), according to t -test. Error bars show standard deviation. Means (black bar) are also indicated. Scale bar 10 µm Full size image In this paper, we have explored the possibility of dosage-driven effects of ZMM genes [32] , [33] in meiotic adaptation to allopolyploidy. We first observed that acquisition of additional copies of ZMM genes by small scale duplications, as exemplified by wheat’s ZIP4 [4] , are exceptional events (Fig. 1 ; Supplementary Figs. 1 – 6 ) and not a convergent phenomenon in plant polyploids. Rather, we found a consistent and rapid reduction of copy number for genes encoding MSH4, MSH5, MER3 and ZIP4 following independent WGDs, while SHOC1 and HEI10 showed higher duplicate retention rates (Fig. 1 ; Supplementary Figs. 1 – 6 ). HEI10 is the only plant ZMM protein known to affect homologous recombination in a dosage-dependent manner, with the number of ZMM-dependent crossovers between homologous chromosomes increasing and decreasing with increased and decreased HEI10 copy number, respectively [33] . The higher HEI10 duplicate retention observed is therefore consistent with the most widely accepted theory that explains the fate of gene duplicates post-WGD and posits that selection to cope with gene dosage constraints contributes to prolonged duplicate retention [34] , [35] . The same theory predicts that “gene duplicates that are not under selection to be retained in duplicate post-WGD are lost at random [35] ”. MSH4 genes, which returned to singletons in all species except the most recent polyploids (Fig. 1 ), may illustrate this second trend. According to some authors, however, such a consistent pattern of gene loss is unlikely to be the result of a purely random and neutral process, but rather suggests duplicates have negative fitness impacts and are actively selected against [14] , [15] , [35] . To gain concrete insights into the consequences of MSH4 duplicate loss, we have interrogated meiosis in recent allotetraploid B. napus when MSH4 duplicates return to single copy. MSH4 accounts for the majority of meiotic crossovers in most organisms, including plants [25] , [26] . We first confirmed that MSH4 plays the same role in B. napus as in other plants: though not required for synapsis completion (Supplementary Fig. 13 ), MSH4 is essential to ensure normal crossover numbers between homologues (Table 1 ; Figs. 2 and 3 ) and, therefore, strictly required to ensure fertility. Most importantly, our results showed that normal levels of homologous crossovers are robust against MSH4 gene duplicate loss even when only one single functional allele of the least expressed copy was present (in the A + A 1 C 1 C 1 plant, Fig. 3 ; Supplementary Figs. 16f and 17f ). Conversely, we showed that crossover formation between homoeologous chromosomes fluctuates in a dosage-sensitive manner. It is maximum when all MSH4 copies are functional, decreases progressively with the number of copies and approximates zero when all MSH4 copies are not functional (Fig. 4 ). Together, our results suggest that MSH4 is in excess during normal meiosis (euploids) but is rate-limiting for allohaploid meiosis. Why does MSH4 become limiting only when crossovers are formed between homoeologous chromosomes in allohaploids? A tentative explanation is that a greater cellular concentration of MSH4 is required to stabilize inherently less stable/more transient early inter-homoeologue recombination intermediates that tend to abort before they mature into crossovers. Future work should test this mechanistic hypothesis. This dispensability of MSH4 duplicates (as long as one functional allele is present) shows that return of MSH4 to single copy is unlikely to induce a selective cost in allopolyploids. Quite the contrary, our results suggest that MSH4 duplicate loss could be beneficial. Providing that inter-homoeologue crossover formation in allohaploids is a good proxy for the situation in the euploids, where both homologues and homoeologues are competing, MSH4 copy number reduction is likely to specifically reduce crossovers between homoeologous chromosomes and thus contribute to improved chromosome segregation. Taken alone, this observation, which is consistent with pervasive MSH4 duplicate loss, would indicate that MSH4 is potentially a “major player” in the meiotic adaptation of allopolyploids. However, combined with the results from wheat (in which ZIP4 is the main actor), they could suggest that modulation of the entire the ZMM pathway, or at least part(s) of it, could contribute to meiotic stabilization in allopolyploids. It is not clear whether MSH4 and ZIP4 act on the same step of the ZMM pathway, or even that their specific role is conserved between species. For example, although no ZMM crossovers can form when either MSH4 or ZIP4 are absent in Arabidopsis [8] , [25] , rice meiosis seems to retain some residual ZMM-dependent events in oszip4 mutant [9] . Likewise, the MSH4-MSH5 heterodimer is thought to act upstream of ZIP4 in rice [26] , [36] , but it seems to be the opposite in yeast [37] . Finally, we do not know why inter-homoeologue crossover suppression results from MSH4 duplicate loss in B. napus (this study) but ZIP4 duplication in wheat [4] . These differences call for further investigation into the effect of the loss/gain of individual ZMM duplicates on crossover formation between homologous and homoeologous chromosomes in recent allopolyploids. This notwithstanding, our results could lead to considering a simple and general route for meiotic adaptations in allopolyploids: i.e., through reduction in the efficiency of the ZMM pathway that would be substantial enough to prevent inter-homoeologue crossover formation but not to compromise the occurrence of (at least) one crossover per homologue (i.e., the obligate crossover). If that is the case, then there would be no need to acquire new meiotic function(s) to sort divergent chromosomes, as the basic machinery would be sufficient to achieve this outcome. In addition, beneficial variants of pre-existing meiotic of genes could occur with greater ease, or in greater proportion, as they would be mainly loss-of-function alleles: e.g., dominant-negative mutations that poison ZMM multiprotein complexes (e.g., MSH4-MSH5 [38] , [39] or MSH5-ZIP4 [37] ) or nonsense / missense mutations that suppress or knock down the function of one gene. In any event, however, our result suggest that reduced cellular availability of MSH4 is unlikely to contribute autopolyploid meiosis stabilization, where the challenge is to prevent multivalent formation between chromosomes with little degree of differentiation. In this context, reducing the absolute number of crossover events, rather than improving their stringency (i.e., homologous vs homoeologous), plays a greater role [40] , [41] , [42] . The invariability of homologous crossover numbers with varying MSH4 copy numbers (Fig. 3 , Supplementary Figs. 16 and 17 ) is not conducive to this process. This difference justifies why genome scans in diploid and autotetraploid Arabidopsis arenosa populations revealed that differentiation (rather than duplicate loss) of structural components of meiotic chromosomes (rather essential factors for ZMM pathway) likely mediates autopolyploid stabilization [41] . To conclude, our results not only shed new light on the longstanding conundrum of meiotic adaptation in polyploids, they also open fruitful avenues towards future applications. These arise from a better understanding of the particular mechanisms that govern recombination between differentiated chromosomes, such as stabilization of synthetic allopolyploids [43] , [44] or manipulating recombination-associated diversity in certain hybrid contexts [45] . Copy number assessment and phylogeny construction We first constructed an orthologous set of ZMM homologous proteins identified from BLASTP and TBLASTN searches against the Non-redundant protein sequences database of NCBI, the predicted protein sequences or current genomes assemblies available in EnsemblPlants ( http://plants.ensembl.org/index.html ), Plaza v4.0 [46] ( https://bioinformatics.psb.ugent.be/plaza/ ), Phytozome v12 ( https://phytozome.jgi.doe.gov/pz/portal.html ), MycoCosm ( https://genome.jgi.doe.gov/programs/fungi/1000fungalgenomes.jsf ) and/or some other website specifically dedicated to a group of related species (e.g. https://solgenomics.net/ ; https://sunflowergenome.org/ ). The sources of the amino acid sequences are provided in Supplementary Data 1 . Gene trees were reconstructed using the Maximum-likelihood (ML) method implemented in the phylogeny pipeline provided by Phylogeny.fr ( http://www.phylogeny.fr/ ) [47] . Multiple alignments were carried out with MUSCLE (full mode). Alignment curation was implemented using GBLOCKS, allowing smaller final blocks and gap positions within the final blocks. Phylogenetic trees were generated using PhyML v3.0 after estimating the Gamma distribution parameters, the proportion of invariables sites and the transition/transversion ratio. The trees were customized and annotated using iTOL ( https://itol.embl.de/ ). The occurrence and age for the past WGDs were taken from refs. [1] , [18] , [19] , [48] , [49] , [50] , [51] , [52] . We used (i) collinearity information (i.e., location within conserved block) as inferred from the WGDotplot applet of PLAZA 4.0 and/or the SynMap applet of the CoGe platform ( https://genomevolution.org/CoGe/SynMap.pl ), (ii) phylogenetic information (using a subset of related proteins) and/or (iii) Ks (i.e., number of synonymous substitutions per synonymous site) estimation to determine whether a gene pair has arisen from a given WGDs [10] . If in doubt, the pair of duplicates was considered as “non-assigned”. Plant material Brassica napus L. cv. Tanto is a double-low spring cultivar obtained at INRA Rennes (France). This is the accession used to develop the RAPTILL EMS population (described in ref. [53] ), in which we looked for mutations in BnaA.MSH4 and BnaC.MSH4 . Microspore culture was performed to isolate allohaploid plants following the protocol detailed in ref. [54] . Microspores were extracted from buds between 3.8 and 4.5 mm in length previously sterilized in bleach and suspended at a density of 100.000 microspores/mL in a modified Lichter’s medium with 0.5 mg/L naphthaleneacetic acid, 0.05 mg N6-benzyladenine, and 13% sucrose and without potato extract. This suspension was incubated 24 h in the dark at 4 °C and, after centrifugation and replacement of the old medium by a fresh one, was incubated on plates in the dark at 30 °C for 14 days during which embryo development takes place. After this period, plates were moved to a slow gyratory shaker (60 rpm) and incubated in the dark at 28 °C for an additional week. After this incubation, embryo germination was induced in B5 liquid medium with 0.1 mg/L gibberellic acid and 1% sucrose incubated on a gyratory shaker (80 rpm) at 25 °C in light for 10 days. Next, the embryos were cultivated in long day greenhouse conditions (see below) on B5 solid medium (0.8% agar) with 0.1 mg/L gibberellic acid and 2% sucrose until root development allowed transference of the plants to soil. Ploidy level verification is recommended as few diploids might have been regenerated. All plants (euploids and allohaploids) were cultivated in standard long day greenhouse conditions (16-hour light/8-hour night photoperiod, at 22 °C day and 18 °C night). Identification of Brassica MSH4 homologues MSH4 homologues were identified by querying the MSH4 coding sequence of A. thaliana (AY646927) against the reference assemblies of B. rapa [55] ( http://brassicadb.org/brad/blastPage.php ), B. oleracea [56] ( http://plants.ensembl.org/Multi/Tools/Blast?db=core ) and B. napus [16] , [57] ( http://www.genoscope.cns.fr/blat-server/cgi-bin/colza/webBlat and http://appliedbioinformatics.com.au/gbrowseblast/cgi-bin/index.pl ). Sequence alignments then confirmed that BnaA.MSH4 / BnaA08g08260D and BnaC.MSH4 / BnaCnng35120D correspond to the two MSH4 genes isolated by previous screening a BAC library from B. napus cv. Darmor-bzh [10] . TILLING We screened the RAPTILL EMS population following exactly the same protocol as described in ref. [53] . Briefly, we targeted a region of 1 Kb of the MutSac domain of BnaA.MSH4 and BnaC.MSH4 . 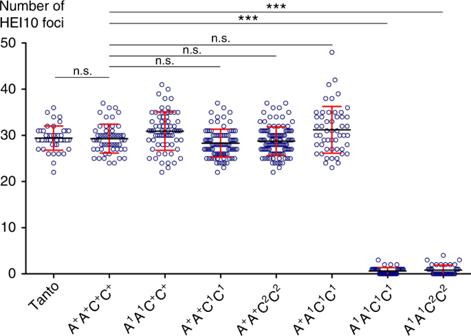Fig. 3 Robustness of ZMM-dependent crossovers toMSH4copy number reduction inB. napuseuploids. Scatter plot of HEI10 (class I crossover) foci in the different genotypes, as determined by HEI10 immunolocalization. *** indicates highly significant variations (p-value < 0.0001) according to Kruskal–Wallis test. Error bars show standard deviation. Means (black bar) are also indicated 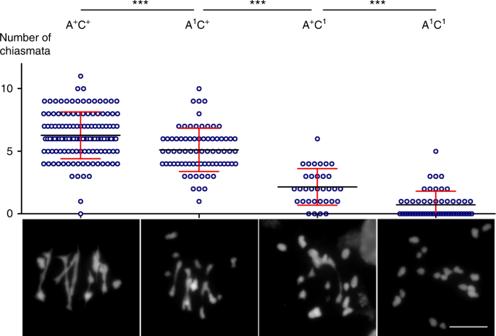Fig. 4 Decreased crossovers uponMSH4copy number reduction inB. napusallohaploids. Scatter plot showing the number of chiasmata estimated for allohaploids carrying varying doses of functional andmsh4mutant alleles. Each genotype is illustrated below with a cytological image as example. N.s indicates non-significant variations whereas *** indicates highly significant variations (p-value < 0.0001), according tot-test. Error bars show standard deviation. Means (black bar) are also indicated. Scale bar 10 µm We used copy-specific primers (T_MSH4AF1, T_MSH4AR1, T_MSH4CF1 and T_MSH4CR1; Supplementary Table 3 ) to amplify BnaA.MSH4 and BnaC.MSH4 separately. The resulting amplicons span the regions between the positions 4144–5126 and 4161–5148 in the genomic sequences of BnaA.MSH4 and BnaC.MSH4 , respectively. The screens for mutations then implemented the PMM (Plant Mutated on its Metabolites) method [58] , [59] . We produced two different F1 hybrids that combined bnaA.msh4-1 (A 1 ), the mutant allele selected for BnaA.MSH4 , with either bnaC.msh4-1 (C 1 ) or bnaC.msh4-2 (C 2 ), the two mutant alleles selected for BnaC.MSH4 . These F1s were self-fertilized to produce segregating F2 progenies among which we selected plants that contained varied number and assortments of Wild Type (A + or C + ) and mutant msh4 alleles (A 1 , C 1 or C 2 ) (Supplementary Fig. 6 ). Genotyping The mutant alleles were identified using cleaved amplified polymorphic sequences (CAPS) assay targeting the causative EMS-SNP. The list of primers and restriction enzymes in given in Supplementary Tables 3 and 4 . Cytological analysis Staged anthers were isolated from fixed buds in ethanol:acetic acid 3:1 (v/v) and used to produce meiotic spreads as described in detail in ref. [60] . Briefly, fixed anthers were firstly rinsed in 10 mM citrate buffer pH 4.5, and incubated by 3.5 h at 37 °C in a digestion mix (0.3% cellulase, 0.3% pectolyase Y23 and 0.3% cytohelicase in citrate buffer pH 4.5). Individual digested anthers were carefully rinsed in water and homogenized in a drop of water placed on a microscopy glass slide. After adding 20 µL of 60% acetic acid the resulting drop was stirred during 4 min on a hot plate at 45 °C to remove the cytoplasm of cells. Finally, the drop was fixed by pipetting etanol:acetic acid (3:1) and allowing the slide to dry before mounting the slide. Chiasma number was estimated on metaphase I spread chromosomes counterstained with 4′,6-diamidino-2-phenylindole (DAPI) based on bivalent shape. Open “rod” bivalents were considered to contain one single chiasma while closed ring bivalents were scored as two (one on each arm). For the study of allohaploids, all scorings were done blindly. Spreads were also used for immunolocalization. Raw counts of bivalent, univalent and chiasma numbers are provided in Supplementary data 2 . Immunolocalization of meiotic proteins Immunodetection of ASY1 and ZYP1 followed the protocol described by ref. [8] that uses fresh anthers treated with 1% lipsol and fixed in 4% paraformaldehyde on a slide. These slides were washed in 0.1% Triton in PBS (PBS-T) and incubated with the corresponding antibodies diluted in 1% BSA at 4 °C for 24 h. Finally, slides were washed in PBS-T were done before mounting with DAPI plus Vectashield. Immunodetection of MLH1, HEI10, REC8 and SCC3 proteins was performed following the protocol described in detail in ref. [61] . This protocol requires a microwave treatment of recently fixed spreads at 850 W in citrate buffer pH 6 that ends by transferring the slides immediately to PBS-T. After this treatment slides followed the antibody incubation and all the successive steps described for standard immunodetection with the difference of a longer antibody incubation (48–72 h). The anti-MLH1 and anti-HEI10 antibodies, both obtained in rabbit serum, were used at dilution 1:200. The antibodies raised against SCC3 and REC8, from guinea pig (GP) and rat serum, respectively, were diluted at 1:250. Anti-ASY1 and anti-ZYP1, obtained in guinea pig (GP) and rabbit, respectively, were both used at dilution 1:500. Secondary antibodies were Alexa488-anti-rabbit (green) and Alexa568-anti-GP and -anti-rat (red). Raw counts of HEI10 foci are provided in Supplementary Data 2 . Fluorescent microscopy All images were obtained using a Zeiss AxioObserver microscope and were analyzed by means of Zeiss Zen software and were organized in panels with Adobe Photosoft CS3. RNA extraction and cDNA obtention RNA was extracted from buds selected by size using RNeasy Mini Kit (Qiagen). One extra step of clean-up and DNAse treatment was added to the extraction protocol. Resulting RNA was utilized for cDNA obtention using RevertAid First Strand cDNA Synthesis Kit (Thermo Fisher Scientific). The presence and absence of cDNA and residual genomic was assessed using the primers Q_UBC21R1, Q_UBC21L1, Q_MSH4F1 and Q_MSH4R1 (Supplementary Table 3 ). Euploid and allohaploid material was sampled simultaneously under the same conditions. Quantitative PCR Three biological replicates were analyzed for every euploid genotype, each replicate being located on a separate qPCR plate. For the allohaploids, a total of five plants were used. Three of them, each representing a distinct genotype, were distributed among three different plates. The last two plants, which represented the same fourth genotype, were distributed on two and one plate, respectively. Three technical replicates were used for all (euploid and allohaploid) plants, all located onto the same plate. We used the ubiquitin gene UBC21 as a reference to normalize the expression of the target MSH4 . The primers used in these experiments (Q_UBC21R1, Q_UBC21L1, Q_MSH4F1 and Q_MSH4R1) are given in Supplementary Table 3 . Variation of MSH4 expression level between genotypes was assessed using an ANOVA with two fixed effects (Genotype and Plate) and the difference in threshold cycle between MSH4 and UBC21 as the dependent variable. Pairwise comparisons of samples after ANOVA were done using post-ANOVA Tukey’s test (alpha = 0.05). Pyrosequencing For pyrosequencing, cDNA and genomic DNA was used to test for amplification bias. The primers utilized were PS_MSH41F (5′-TGCTCAGATTGGCTGCTATGT-3′) as forward primer, PS_MSH4R (5′-TTCTTGTGAATATGCGGTCAAC-3′) as reverse primer and PS_MSH4S (5′-CAACCACACGCATAGT-3′) as sequencing primer. Pyrosequencing reaction was performed with PyroMark Q24 v2.0.6 (Qiagen). Reporting summary Further information on research design is available in the Nature Research Reporting Summary linked to this article.